The role of charge-transfer states in energy transfer and dissipation within natural and artificial bacteriochlorophyll proteins Understanding how specific protein environments affect the mechanisms of non-radiative energy dissipation within densely assembled chlorophylls in photosynthetic protein complexes is of great interest to the construction of bioinspired solar energy conversion devices. Mixing of charge-transfer and excitonic states in excitonically interacting chlorophylls was implicated in shortening excited states’ lifetimes, but its relevance to active control of energy dissipation in natural systems is under considerable debate. Here we show that the degree of fluorescence quenching in two similar pairs of excitonically interacting bacteriochlorophyll derivatives is directly associated with increasing charge-transfer character in the excited state, and that the protein environment may control non-radiative dissipation by affecting the mixing of charge-transfer and excitonic states. The capability of local protein environments to determine the fate of excited states, and thereby to confer different functionalities to excitonically coupled dimers substantiates the dimer as the basic functional element of photosynthetic enzymes. The effective capture of incoming light is critical to the efficiency of all solar energy conversion systems. Regardless of specific architecture, any system must maintain sufficient photon throughput to keep up with the formation rates of its end products. At the same time, it must be robust to the large fluctuations of solar intensity during the day. In natural photosystems, most of the incident light is absorbed by well-organized and densely packed arrays of chlorophylls (Chls) or bacteriochlorophylls (BChls) within light-harvesting protein complexes (LHCs). From there, the excitation energy is transferred rapidly and efficiently to reaction centre (RC) proteins where a few (B)Chls and other redox cofactors drive charge separation and the ensuing chemistry [1] , [2] , [3] , [4] . The particular arrangement of pigments within the LHCs, and their specific protein environment prevent much of the non-radiative energy dissipation processes that prevail in highly concentrated (B)Chl solutions [5] . This enables the assembly of highly absorbing (B)Chl arrays without compromising the efficiency of energy transfer to the RCs. It was recently proposed that the protein environment not only holds the pigments at certain orientations but also has the ability to switch energy dissipation on and off, thereby actively regulating the photon fluxes through the RC [6] , [7] , [8] . This hypothesis and the molecular mechanisms of a variety of regulatory energy dissipation processes collectively known as non-photochemical quenching (NPQ) are subjects of considerable debate [9] , [10] . Particularly, LHCs contain carotenoids that are clearly involved in NPQ [8] , [10] , [11] , [12] , [13] , but evidence of non-radiative quenching that does not require any carotenoids both in LHC antenna and in Chl–Chl pigment arrangements [14] , [15] have led to much controversy over the role of dissipation by (B)Chl pairs in NPQ in vivo [16] , [17] , [18] . Charge-transfer (CT) states between two neighbouring (B)Chls are most likely involved in non-radiative energy dissipation. Their formation is inevitable in excitonically coupled (B)Chl pairs [19] , [20] , but the yields of formation, and whether or not they provide effective non-radiative relaxation pathways critically depend on their coupling to the excited and ground states, which in turn depends on the protein environment of the pairs. However, the detailed conditions that will either prevent or induce non-radiative quenching by CT states are yet unclear. In this work we explore the means of controlling CT states within a protein environment by comparing two simple protein systems that contain very similar pairs of excitonically coupled (B)Chls but that differ significantly in their levels of fluorescence quenching. The first is an artificial system that was recently established by one of us [21] ; it is comprised of two or three water-soluble zinc-substituted BChl derivatives (ZnBChlide) incorporated into HP7, a de novo designed protein four-helix bundle that was originally planned for haem binding [22] . The excitonic interactions within the HP7-bound ZnBChlide pair were found to drastically quench fluorescence [21] . By contrast, the second system, the B820 subunit of the purple bacterial LH1 complex is a minimal functional subunit of a natural system. Thus, it keeps the quenching of its pair of excitonically coupled BChls to a level that will still allow efficient energy transfer among the subunits of the native LH1 complex. We employ Stark absorption and fluorescence (SA and SF, respectively) spectroscopy for monitoring the formation of CT states in the photoexcited BChl pair of B820, and ZnBChlide pairs bound to either HP7 or its single-histidine knockout variant HP7H7F. Comparing the Stark spectra of the natural and artificial systems provides us with valuable insights into the role of CT states in relaxation pathways of excitonically coupled (B)Chls. Absorption and SA spectra of ZnBChlide in HP7 and HP7H7F A previous study has rigorously characterized the binding of ZnBChlide to HP7 and HP7H7F by a series of absorption and circular dichroism (CD) spectroscopic titrations [21] . These revealed a stepwise binding equilibrium of ZnBChlide to specific protein-binding sites, and clearly distinguished between the monomeric form of protein-bound ZnBChlide that was predominant at substoichiometric ZnBChlide:protein ratios, and the excitonically coupled dimer form that emerged upon exceeding the 1:1 molar ratio. Notably, the saturation point was also clearly observed because binding ZnBChlide to HP7 or HP7H7F leads to significant red shifts of ZnBChlide’s Qx and Qy absorption bands from 569 nm and 764 nm in the free pigment to 593 nm and 773 nm in the protein-bound pigment, respectively [21] . In this work, we wanted to compare the monomeric and dimeric forms of ZnBChlide. On the basis of the previous work, we prepared substoichiometric samples of low (1:3) ZnBChlide:protein molar ratios, and saturated samples of 2:1 and 3:1 ZnBChlide:HP7 and ZnBChlide:HP7H7F molar ratios, respectively. As expected, the absorption and CD spectra ( Supplementary Fig. 1 ) of the saturated samples were typical of excitonically coupled ZnBChlide dimer featuring a characteristic split of the Qy absorption into a highly absorbing low-energy exciton absorption band and a weakly absorbing high-energy exciton absorption band around 810 and 760 nm, accompanied by positive and negative CD bands, respectively. There was no indication of free ZnBChlide in the HP7 sample, but a minor fraction of unbound ZnBChlide was observed in the saturated HP7H7F sample as indicated by the 575-nm shoulder in the Qx absorption band. We estimate this fraction to be <10% of the total pigments in the sample. In the substoichiometric samples, all the ZnBChlide was bound to the protein and the monomeric form was predominant; however, since the total complex concentrations were >100-fold higher than the dissociation constants of dimeric ZnBChlide, there were already significant populations of this form in the substoichiometric samples. These were obvious in the emergence of low-energy exciton absorption bands, and typical split CD spectra in the substoichiometric samples. The Qy absorption band of dimeric ZnBChlide emerged as a shoulder around 800 nm next to the peak of the monomeric form at 768 nm in the absorption band of the HP7–ZnBChlide complex. It was even more pronounced in the HP7H7F–ZnBChlide sample, where it led to a broad asymmetric band centred at 790 nm ( Fig. 1a ). 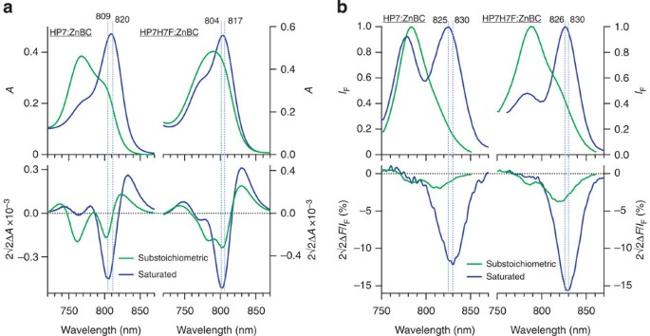Figure 1: Absorbance and fluorescence with respective Stark spectra of HP7– and HP7H7F–ZnBChlide complexes. (a) Absorbance and SA spectra of substoichiometric and saturated complexes recorded at 77 K. Dashed lines mark the absorption peaks (derived from 2nd derivative analysis) of the lowest exciton bands of the substoichiometric and saturated samples. (b) Fluorescence and SF spectra of substoichiometric and saturated complexes recorded at 77 K. The SF spectra were normalized to the fluorescence intensity at the highest peak maximum. Dashed lines mark emission peaks and SF-negative peaks of the lowest exciton bands of the saturated samples. Figure 1: Absorbance and fluorescence with respective Stark spectra of HP7– and HP7H7F–ZnBChlide complexes. ( a ) Absorbance and SA spectra of substoichiometric and saturated complexes recorded at 77 K. Dashed lines mark the absorption peaks (derived from 2nd derivative analysis) of the lowest exciton bands of the substoichiometric and saturated samples. ( b ) Fluorescence and SF spectra of substoichiometric and saturated complexes recorded at 77 K. The SF spectra were normalized to the fluorescence intensity at the highest peak maximum. Dashed lines mark emission peaks and SF-negative peaks of the lowest exciton bands of the saturated samples. Full size image The SA spectra associated with the Qy bands featured derivative-like lineshapes. The zero-crossing points for each SA spectrum were significantly shifted from the respective absorption peak indicating the simultaneous contributions from zero-, first- and second-order derivatives to the SA lineshape. In general, the Stark effects associated with the low-energy exciton bands were much more significant than those associated with the shorter wavelength bands. This was most pronounced in the SA spectra of the substoichiometric samples, whereby the short- and long-wavelength SA bands had similar intensities despite the smaller contribution of the latter to the corresponding absorption spectra. The spectra of the saturated samples were similar in lineshape and peak positions to previously recorded SA spectra of the B820 subunit [23] . Fluorescence and SF spectra of ZnBChlide in HP7 and HP7H7F Similar to the absorption, the fluorescence spectra of substoichiometric and saturated HP7– and HP7H7F–ZnBChlide complexes ( Fig. 1b ) appeared to be comprised of two emission bands. One band, at 780 nm was predominant in the substoichiometric samples, whereas the other band appeared as a shoulder around 820 nm in the substoichiometric samples and became the strongest band in the saturated samples. Thus, it is reasonable to assign the first band to protein-bound ZnBChlide monomers, and the second to the low-energy exciton of ZnBChlide dimers. The fluorescence from the dimers is strongly quenched; hence the available emissive monomers contribute significantly to the emission spectra of the saturated samples although their concentrations are much lower than the dimers. Notably, since the samples were excited between 600 and 610 nm, it is unlikely to expect any contribution to the fluorescence from unbound ZnBChlide that hardly absorbs in this region. In contrast to the derivative-like lineshapes of SA bands, the lineshapes of the SF bands resembled inverted fluorescence emission bands whose peaks were red shifted by about 5 nm with respect to the fluorescence emission peaks. The apparent similarity to the shape of the fluorescence spectrum, and the large negative amplitude indicate that the major component of the SF spectrum is the zero-order-derivative contribution (ZDC), which reflects the field-induced reduction of the fluorescence intensity (FIRFI). The SF bands associated with the low-energy exciton fluorescence were already predominant in the spectra of the substoichiometric complexes despite the minor contribution of the low-energy exciton to the overall fluorescence spectra, and became about fivefold more intense in the saturated samples. This suggests that the field effects on the low-energy exciton emission bands were very large and much more pronounced than on the ZnBChlide monomer emission bands. Electro-optic parameters from SA and SF spectra To gain more insight into the origin of the Stark effects, and estimate the electro-optic molecular parameters, the experimental data were analysed on the basis of the standard Liptay formalism [24] , [25] , [26] . Each absorption and fluorescence spectrum was modelled as the sum of two skewed Gaussian bands, and the respective SA and SF spectra were constructed from the weighted superposition of the zero-, first- and second-order Stark derivative of each band. Implementing the model in a global curve-fitting algorithm resulted in good simultaneous fits to the experimental data. Analysis of the absorption and SA spectra ( Fig. 2 ) clearly indicated that second derivatives had the greatest contribution to the SA spectral lineshapes, and the contribution of zero-order derivatives to the lower-energy band was close to zero. The analysis thus yielded significant magnitudes of Δ μ for all the SA bands, and negligible ZDC to the low-energy band ( Table 1 ) of each SA spectrum. The magnitudes of Δ μ ranged from 2.2 to 4.3 D / f , which is similar to the values derived from SA spectra of the natural purple bacterial B820 complex [23] . 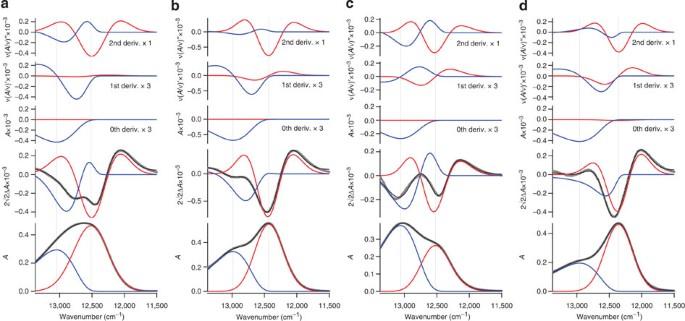Figure 2: Curve-fitting analysis of absorption and SA spectra. (a) Substoichiometric HP7H7F, (b) saturated HP7H7F, (c) substoichiometric HP7, (d) saturated HP7. Spectra were simultaneously fitted with two skewed Gaussian bands shown in red and blue. Experimental data are shown in grey dots, and the fitted curves in solid black lines. The top three graphs present the zero-, first- and second-order derivative components of the SA spectra of each band. For better comparison theyscale was kept constant and the scaling factors applied to each component are listed on each graph. Figure 2: Curve-fitting analysis of absorption and SA spectra. ( a ) Substoichiometric HP7H7F, ( b ) saturated HP7H7F, ( c ) substoichiometric HP7, ( d ) saturated HP7. Spectra were simultaneously fitted with two skewed Gaussian bands shown in red and blue. Experimental data are shown in grey dots, and the fitted curves in solid black lines. The top three graphs present the zero-, first- and second-order derivative components of the SA spectra of each band. For better comparison the y scale was kept constant and the scaling factors applied to each component are listed on each graph. Full size image Table 1 Molecular parameters estimated from SA and SF analyses. Full size table The curve-fitting analysis of fluorescence and SF spectra ( Fig. 3 ) emphasized the exceptionally strong FIRFI of the long-wavelength bands in the SF spectra ( Table 1 ). The estimated magnitudes of Δ μ ranged from 2.4 to 4.8 D / f , which is very similar to the values obtained from SA spectra. 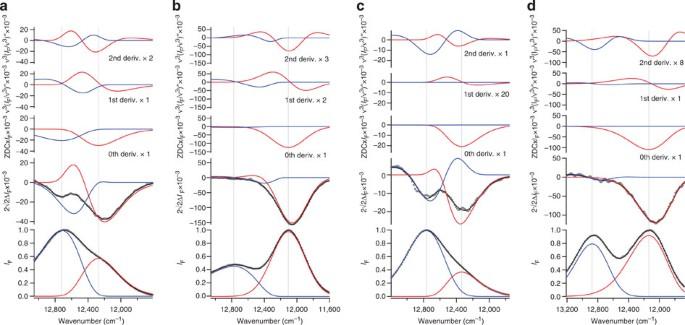Figure 3: Curve-fitting analysis of fluorescence and SF spectra. (a) Substoichiometric HP7H7F, (b) saturated HP7H7F, (c) substoichiometric HP7, (d) saturated HP7. Spectra were simultaneously fitted with two skewed Gaussian bands. Line colours and markers are the same as inFig. 2. Figure 3: Curve-fitting analysis of fluorescence and SF spectra. ( a ) Substoichiometric HP7H7F, ( b ) saturated HP7H7F, ( c ) substoichiometric HP7, ( d ) saturated HP7. Spectra were simultaneously fitted with two skewed Gaussian bands. Line colours and markers are the same as in Fig. 2 . Full size image Comparison of artificial and natural BChl–protein complexes The absorption and SA spectra of the artificial ZnBChlide complexes of HP7 and HP7H7F were very similar to previously published spectra of the B820 subunit of LH1 from the carotene-free purple bacteria strain Rhodospirillum Rubrum G9+, a natural light-harvesting system that contains a similar dimer of BChls [23] , [27] . Our measurements of fluorescence and SF spectra of the natural system revealed a high degree of similarity to saturated HP7 and HP7H7F complexes ( Fig. 4 ). Particularly, all the samples featured an emission band around 820 nm with a dominant-negative SF band that was slightly red shifted. However, the Stark effect on the 820-nm band of the natural B820 complex was more than threefold smaller than the effect on the analogous band in the artificial complexes. This was also reflected in the magnitude of ZDC in B820 that was about half the magnitude of saturated HP7 and HP7H7F. Interestingly, the change in polarizability, Δ α , of the low-energy exciton band was negative both in the artificial and the natural complexes. The emission band at 780 nm observed in the B820 sample originates from a fraction of protein-bound monomeric BChl species known as B777 that is at equilibrium with the B820 dimeric BChl species [23] . Similar to the monomeric ZnBChlide species in the HP7 and HP7H7F samples, B777 species are more emissive than the low-energy excitonic bands and thereby contribute significantly to the fluorescence spectra despite their apparent low concentration (see Supplementary Fig. 2 for B820 absorption spectra). As expected, the SF from these monomeric species was negligible compared with the respective signal from the dimeric species. 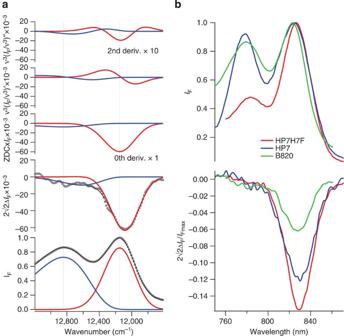Figure 4: Fluorescence and SF spectra ofRs. RubrumG9+ LH1 B820. (a) Curve-fitting analysis. Spectra were simultaneously fitted with two skewed Gaussian bands. Line colours and markers are the same as inFig. 2. (b) Normalized fluorescence and SF emission spectra of saturated HP7H7F and HP7, and the B820 subunit. Figure 4: Fluorescence and SF spectra of Rs. Rubrum G9+ LH1 B820. ( a ) Curve-fitting analysis. Spectra were simultaneously fitted with two skewed Gaussian bands. Line colours and markers are the same as in Fig. 2 . ( b ) Normalized fluorescence and SF emission spectra of saturated HP7H7F and HP7, and the B820 subunit. Full size image Our measurements reveal that the SA and SF spectra of excitonically coupled ZnBChlide dimers within the HP7 and HP7H7F protein complexes are characterized by a highly absorbing low-energy exciton state that features considerable changes of dipole moment (Δ μ ) accompanied by a large negative change in polarizability (Δ α ) following excitation and subsequent fluorescence; in addition, the fluorescence from this exciton state exhibits very large FIRFI. The large values of Δ μ that were derived from the SA spectra were similar to previously published values of BChl dimers in purple bacterial LH complexes [23] . These were explained in terms of mixing an intradimer CT state with the low-energy exciton state [28] . The similar Δ μ values obtained from the SF spectra imply that the CT character of the Frank–Condon excited state of ZnBChlide dimer is maintained in the vibrationally relaxed low-energy exciton state from which light is eventually emitted by fluorescence. By contrast, the ZDCs were negligible in the low-energy exciton SA bands, but very large and negative in the respective SF bands. Therefore, the observed exceptionally strong FIRFI reflected by the negative ZDC values, particularly in the saturated complexes, may be caused by field-induced modulation of either the fluorescence transition moment, or the rates of non-radiative relaxation processes. Since the negligible ZDC values of the SA spectra indicate that the absorption transition moments were hardly changed by the electric field, it is likely to assume that the respective fluorescence transition moments are not significantly affected. Thus, the large FIRFI values probably indicate the acceleration of non-radiative relaxation processes by the applied electric field. Furthermore, the FIRFI in the SF spectra of the dimeric species were about twofold larger in the saturated than in the substoichiometric complex, and hence appeared to be correlated with the extent of excitonic interaction within the dimeric ZnBChlide and with the extent of fluorescence quenching. We observed a similar trend in a SF study of LHCII of higher plants, where the FIRFI magnitude of the excitonic emission was found to increase remarkably upon induction of quenching [29] . The much lower FIRFI in the natural functional B820 subunit with respect to its highly quenched artificial analogue, HP7, is most revealing and underpins the role of mixing CT and excitonic states in controlling fluorescence quenching. Mixed exciton/CT states have been implicated in the regulation processes of non-radiative relaxation of excited states in photosynthetic light-harvesting systems [17] , [18] , [29] , [30] . Here, we observe a direct correlation between the CT character of the excited state of excitonically coupled BChl pairs and its non-radiative dissipation. The close similarity between all other absorption and emission properties suggests that ZnBChlide in HP7, and BChl in B820 form very similar dimers; hence the marked difference in CT character is most likely due to the effect of the protein environment. Although a molecular structure of the HP7–ZnBChlide is not available, it is likely to assume that the bound pigments are more exposed to the aqueous polar environment than in the transmembrane B820 subunit. This polar environment may stabilize a CT state and improve its coupling to the ground state thereby leading to efficient non-radiative relaxation pathways of the photoexcited ZnBChlide pair. From an evolutionary perspective, the ability to control the CT character of photoexcited Chl and BChl pairs by changing their local protein environment is an elegant and effective means of conferring different functionalities to the same or very similar cofactors. Chl and BChl pairs are commonly used in photosynthetic pigment-proteins, not only for excitation energy transfer but also for initiating photoinduced charge separation. The contribution of CT states to the primary charge separation in purple bacterial RCs was shown by Boxer [31] . More recent and rigorous studies of native and mutant PSII RC revealed that the degree of mixing between exciton and CT states determines the quantum yield of radical pair formation and thereby the efficiency of charge separation [28] , [32] . By combining these insights with the results from this work, we can construct a simple state diagram ( Fig. 5 ) that provides a general mechanism for controlling the fate of photoexcited states in (B)Chl pairs. Assuming very rapid vibrational relaxation from the Franck–Condon singlet excited state to an exciton state that is mixed with a CT state, the level of mixing and hence the CT character of the new state depends on the relative energy levels and coupling constants of the latter two states. Local and external fields are likely to affect the energy of the CT state and its coupling to the exciton state. Similarly, depending on relative energy levels and coupling constants, the exciton/CT state may relax either to the ground state or to a full-charge-separated state that is a real observable state where one molecule in the dimer is one-electron deficient, and the other has an extra electron. These relaxation processes compete effectively with radiative relaxation of the exciton state. Thus, the fate of an excitation may be determined by controlling the relative energy level of the CT state with respect to the ground, photoexcited singlet, and charge-separated states, and its electronic coupling to these states. This mechanism establishes the excitonically coupled dimer of (B)Chls as the primary functional element of the photosystem. As demonstrated here, the protein environment has the means of controlling the fate of excitation by changing the electric fields around a dimer, which makes it a versatile component that can be used for light-induced charge separation, energy transfer and dissipation. 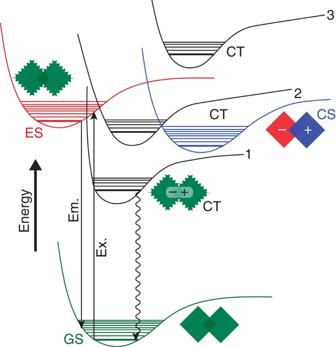Figure 5: Controlling the fate of excitation in excitonically coupled (B)Chl dimers. The photoexcited state of a (B)Chl dimer may exhibit variable CT character according to the mixing of the excitonic state (ES—red potential curve) with a CT state (CT—black potential curves). The fate of excitation may thus be determined by controlling the energies and electronic coupling of the CT state with respect to the exciton state and the ground state (GS—green potential curve). The first scenario (1), results in energy dissipation since the low-lying CT state is coupled to the excited state and provides effective non-radiative relaxation pathways (wiggled arrow) to the ground state. In the second scenario (2), a charge-separated state (CS—blue potential curve) is coupled to the CT state, which leads to charge separation. In the third scenario (3), the CT state is inaccessible because it lies at a higher energy than the excited state and does not compete with radiative relaxation (Em.) from the exciton state. Consequently, the excited state lifetime remains long enough to allow effective excitation energy transfer to neighbouring pigments. Figure 5: Controlling the fate of excitation in excitonically coupled (B)Chl dimers. The photoexcited state of a (B)Chl dimer may exhibit variable CT character according to the mixing of the excitonic state (ES—red potential curve) with a CT state (CT—black potential curves). The fate of excitation may thus be determined by controlling the energies and electronic coupling of the CT state with respect to the exciton state and the ground state (GS—green potential curve). The first scenario (1), results in energy dissipation since the low-lying CT state is coupled to the excited state and provides effective non-radiative relaxation pathways (wiggled arrow) to the ground state. In the second scenario (2), a charge-separated state (CS—blue potential curve) is coupled to the CT state, which leads to charge separation. In the third scenario (3), the CT state is inaccessible because it lies at a higher energy than the excited state and does not compete with radiative relaxation (Em.) from the exciton state. Consequently, the excited state lifetime remains long enough to allow effective excitation energy transfer to neighbouring pigments. Full size image Preparation of protein samples The preparation of ZnBChlide (13 2 -hydroxy-zinc-bacteriochlorophyllide), HP7 and HP7H7F were as previously described [21] . For assembling the ZnBChlide complexes, purified proteins were dissolved in 50 mM HEPES, 1 M NaCl, pH 8.0 buffer to which highly concentrated methanolic ZnBChlide solutions were added. Two distinct ZnBChlide–protein complexes were prepared for HP7 and HP7H7F. A substoichiometric complex was prepared by adding ZnBChlide to a protein:pigment ratio of 3:1, and a saturated complex was prepared by adding ZnBChlide to a protein:pigment ratio of 1:3 in HP7, and 1:2 in the other variants. The samples were concentrated by ultrafiltration on Vivaspin (GE healthcare) 3000 molecular weight cutoff centrifugal concentrators to an optical intensity of 1.5 at 770 nm in a 0.1-mm cuvette. Then, glycerol was added to each sample to a final concentration of 60% (v/v) to produce transparent glasses upon freezing the samples at 77 K. B820 subunit samples were prepared by treating native LH1 complexes isolated from chromatophores of the carotene-free purple bacteria strain R. Rubrum G9+ with n -Octyl-β- D -glucopyranoside, and purifying by size-exclusion chromatography as previously described [27] . Stark spectroscopy SA and SF measurements were performed at 77 K. The stark cell was prepared by placing a drop of the liquid sample between two glass slides coated with indium tin oxide electrodes on their inner surfaces, separated by and glued together with double-sided 110-μm-thick sticky tape. The cell was placed inside the liquid N 2 chamber of an optical cryostat (Oxford Instruments, DN1704). The SA/SF spectrometer was a homebuilt setup, similar to previously described systems [25] , [29] , [33] . Briefly, the excitation wavelength is selected by dispersing the white light continuum of a tungsten-halogen lamp (100 W) through a monochromator (1,200 g mm −1 grating blazed at 350 nm) with 2-mm slit width. The excitation beam is then horizontally polarized upon passing through a Glan-Taylor polarizer and finally hits the sample at an angle of 45°. A sufficiently high sinusoidal a.c. voltage with modulation frequency ω (312 Hz for SA and 80 Hz for SF) is applied to the sample and both SA/SF and absorption/fluorescence signals are recorded simultaneously by a lock-in amplifier (SR850) at 2 ω . The low-distortion sinusoidal a.c. signal is synthesized digitally in the lock-in amplifier, which is ultimately fed to a high-voltage generator to obtain the desired amplification prior applying to the sample. The recorded SA/SF signal is multiplied by 2√2 to convert it to an equivalent d.c. voltage, and finally the SA/SF spectrum is obtained by plotting the SA/SF signal as a function of wavelength ( λ ). The absorption/fluorescence signals of the protein samples are also measured separately at ω with the same lock-in amplifier by locking it to the frequency of an external mechanical chopper at 312/80 Hz. SA spectra were measured at magic angle ( χ =54.7°) at field strength of 0.26 MV cm −1 . SF spectra were recorded at different field strengths ranging from 0.30 to 0.50 MV cm −1 , but for the sake of easier comparison, the spectra were scaled to field strength of 1 MV cm −1 . In addition, all the SF spectra are normalized to the fluorescence intensity at the peak maximum. The excitation wavelengths for the fluorescence measurements were set between 600 and 610 nm region where the corresponding SA signal is almost zero to avoid interference from SA signals. Data analysis The analysis of SA and SF spectra was based on the standard Liptay formalism whereby Δ A ( ν ), the SA intensity at a given energy ν , is expressed as the weighted sum of the zero-, first- and second-order derivatives of the absorption spectrum A [24] , [25] : where F ext is the externally applied electric field, χ is the experimental angle between the direction of F ext and the electric vector of the excitation light and f is the internal field correction factor, which relates the magnitude of the field present at the chromophores to F ext . The ZDC, which reflects the direct effect of the externally applied electric field on the transition moment of the molecule is given by the product ( f F ext ) 2 A χ . The weighting constants B χ and C χ are related to Δ μ and Δ α , the respective differences in electric dipole moment and molecular polarizability between the ground and excited states [25] : where h and c are Planck’s constant and the speed of light, respectively. Since it is very difficult to map precisely the dielectric landscape inside the protein cavity, it is hard to quantify the field correction, f , for the protein, and therefore the experimental values of Δ μ and Δ α are reported in units of (Å 3 / f 2 ) and ( D / f ) ( Table 1 ). By analogy to the SA, the SF intensity, Δ I F ( ν ), is given by The weighting constants B′ χ and C′ χ are given by equations (2) and (3), substituting the differences in polarizability (Δ α ) and dipole moment (Δ μ ) between the emissive state and the ground state, respectively. The ZDC, given by ( f F ext ) 2 A′ χ , reflects the field-induced change in fluorescence intensity arising from the field-induced change in transition moment and/or in the non-radiative process. To obtain the molecular electronic parameters ZDC, Δ α , Δ μ from the absorption and SA spectra each ZnBChlide absorption band was estimated by a skewed Gaussian function where A 0 , ν 0 , σ and b are amplitude, peak position, width and skewness parameters of the skewed Gaussian, respectively. The absorption and SA spectra were assumed to be the weighted sum of skewed Gaussian bands and their analytical derivatives, respectively. More specifically, the Qy absorption band of ZnBChlide was simulated by a weighted sum of two skewed Gaussians. A global-fitting algorithm implemented in the Igor Pro (Wavemetrics Inc.) software was used to simultaneously fit this weighted sum to the experimental absorption, and the weighted sum of the derivatives according to equation (1) to the experimental SA, whereby the parameters ν , σ and b of each band were used as global-fitting parameters common to the absorption and SA data sets. The fluorescence and SF spectra were fitted using the same procedure substituting I F ( ν ) for A ( ν ) in equation (5), and using equation (4) instead of equation (1). How to cite this article: Wahadoszamen, Md. et al. The role of charge-transfer states in energy transfer and dissipation within natural and artificial bacteriochlorophyll proteins. Nat. Commun. 5:5287 doi: 10.1038/ncomms6287 (2014).